Aligned Fe2TiO5-containing nanotube arrays with low onset potential for visible-light water oxidation There remains a pressing challenge in the efficient utilization of visible light in the photoelectrochemical applications of water splitting. Here, we design and fabricate pseudobrookite Fe 2 TiO 5 ultrathin layers grown on vertically aligned TiO 2 nanotube arrays that can enhance the conduction and utilization of photogenerated charge carriers. Our photoanodes are characterized by low onset potentials of ~0.2 V, high photon-to-current efficiencies of 40–50% under 400–600 nm irradiation and total energy conversion efficiencies of ~2.7%. The high performance of Fe 2 TiO 5 nanotube arrays can be attributed to the anisotropic charge carrier transportation and elongated charge carrier diffusion length (compared with those of conventional TiO 2 or Fe 2 O 3 photoanodes) based on electrochemical impedance analysis and first-principles calculations. The Fe 2 TiO 5 nanotube arrays may open up more opportunities in the design of efficient and low-cost photoanodes working in visible light for photoelectrochemical applications. How to find practical techniques for producing clean and sustainable energy is a globally demanding challenge due to the shortage of fossil fuels and global climate changes [1] , [2] . Especially, semiconductor photocatalysis has been widely studied as a promising method for converting sunlight into electricity or fuels and for purifying air and water [3] , [4] , [5] . The efficient solar-to-chemical energy conversion across a wide range of solar spectrum is believed to be important for practical uses of solar-driven clean energy systems [6] . However, for the most of stable metal oxides semiconductor photoanodes such as TiO 2 and ZnO, only ultraviolet light irradiation can be absorbed. Although some semiconductor photoanodes such as Fe 2 O 3 were reported to be able to absorb visible lights, their photocarrier utilization for oxidizing water is relatively low and their quantum efficiencies are usually lower than 10% at 1.23 V versus reversible hydrogen electrode (RHE) [7] , [8] . The architecture of vertically aligned nanotube arrays has shown considerate improvements to the quantum efficiencies of TiO 2 and Fe 2 O 3 photoanodes [9] , [10] , [11] , [12] , [13] , [14] , but the total conversion efficiency of visible lights is still not satisfactory. Therefore, it is highly desirable yet challenging to find an efficient photoanode semiconductor that is capable of using the abundant visible lights. The key to maximize solar energy utilizations in photoanodes is the efficient separation and transportation of visible-light-induced charge carriers in the water-splitting process. There are several remarkable factors that prevent the successful separation and transportation of charge carriers. First, for most of narrow bandgap metal oxide photoanodes, their conduction band minimum (CBM) positions are usually positive versus RHE. A large external electric field energy is therefore needed for the effective charge carrier separation and water-splitting reaction. Second, the depletion region is not long enough to separate the photoexcited carriers in the nanoscale photoanode, leading to a high recombination probability of photocarriers [15] . As a result, the photocarriers are localized within the photoelectrode interior and they can hardly migrate to surface water redox reaction sites [16] , [17] . All these factors significantly undermine the energy conversion efficiency under visible light illumination. Consequently, the development of new strategies that overcome the above limitations and the realization of efficient visible light conversion in narrow-bandgap semiconductor photoanodes are highly in demand. In this work we report for the first time a pseudobrookite iron titanate Fe 2 TiO 5 ultrathin layer supported on TiO 2 nanotube-arrayed photoanode for realizing highly efficient visible light conversion. Fe 2 TiO 5 is a narrow bandgap semiconductor of ca . 2.2 eV with the valence band edge surpassing the water oxidation level [18] . In particular, the CBM of Fe 2 TiO 5 lies nearly at the same energy level as that of TiO 2 , leading to a quick onset of photocurrent under visible light irradiations. Moreover, the electronic and atomic structures of Fe 2 TiO 5 match well with TiO 2 and this would allow a good separation of the photogenerated hole carriers on the hybridized interface. In our design, the Fe 2 TiO 5 layer is sandwiched between TiO 2 and Co ox layers (Co ox layer is coated as the surface catalyst [19] , [20] ). We adopt the vertically self-organized nanotube array for this new photoanode, because it has the unique charge transport property and huge specific surface areas, by taking advantages of Fe 2 TiO 5 and TiO 2 layers with high catalytic efficiencies. The growth of the lattice-matched Fe 2 TiO 5 on TiO 2 is achieved by annealing the TiO 2 /Fe 2 O 3 composite, where a solid-state reaction between Fe 2 O 3 and TiO 2 occured [21] . This closely contacting Fe 2 TiO 5 composite nanotube array guarantees a substantial visible light absorption and introduces hole–electron separation interfaces required for fast separation and effective transportation of the electron–hole pairs. Therefore, our designed system is characterized by high quantum efficiencies (absorbed photon-to-current efficiency (APCE) >40%) under visible lights in the 400–600 nm wavelength range. It may also provide more insights to the optimization of photoelectrochemical performance of oxide semiconductor photoanodes. Structural identification First of all, the as-designed composite photoanode is schematically presented in Fig. 1a–c . Figure 2a–c show the scanning electron microscopy and transmission electron microscopy (TEM) of the system. 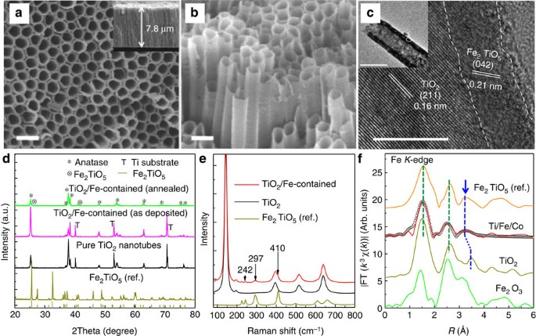Figure 2: Morphology and structural properties of the samples. (a,b) Scanning electron microscopy and and (c) high-resolution TEM images for TiO2/Fe-contained/Cooxnanotube arrays. Scale bars, 200, 200, 5 and 100 nm, (a,b,cand inset ofc, respectively). (d) X-ray diffraction patterns for pure TiO2, Fe2TiO5reference sample and as-deposited TiO2/Fe-contained nanotube arrays, and grazing incidence X-ray diffraction patterns for the annealed TiO2/Fe-contained nanotube arrays. The standard card (PCPDF 76-1158) for orthorhombic Fe2TiO5is shown for reference. (e) Raman spectra for TiO2, TiO2/Fe-contained nanotube-arrayed photoanodes and reference Fe2TiO5(ref.). (f) FeK-edge EXAFS FTs ofk3χ(k) functions for TiO2/Fe-contained/Coox. The empty circles show the fitting results. The FeK-edge spectra for Fe2O3and TiK-edge spectra for TiO2and Fe2TiO5(ref.) are shown for comparison. The reference Fe2TiO5(ref.) sample ind,eandfwas synthesized by solid-state reaction method. It is evident that the nanotube arrays are well-aligned and perpendicular to the underlying substrate, with the tube length and wall thickness of about 7.8 μm and 10 nm, respectively. The morphology and performance of the TiO 2 nanotube substrate were optimized before their modification (see Supplementary Figs 1 and 2 , Supplementary Tables 1 and 2 ). The Fe-containing ultrathin layer can be clearly seen from an area of about 2–3 nm in width near the surface of the composite nanotubes in the high-resolution TEM image ( Fig. 2c and Supplementary Figs 3 and 4 ). The grazing incidence X-ray diffraction patterns for the TiO 2 /Fe-contained/Co ox sample suggest a main anatase structure ( Fig. 2d ). More importantly, new diffraction peaks at 26° and 42° are observed, which can be indexed to the (110) and (042) planes of pseudobrookite Fe 2 TiO 5 , respectively. Furthermore, the lattice space of 0.21 nm corresponding to (042) plane of orthorhombic Fe 2 TiO 5 is observed from the high-resolution TEM image ( Fig. 2c ), in agreement with the selected area electron diffraction patterns ( Supplementary Fig. 5 ). This can be further confirmed by the Raman spectra in Fig. 2e showing three peaks at 242, 297 and 410 cm −1 , among which the 410 cm −1 peak is the strongest. 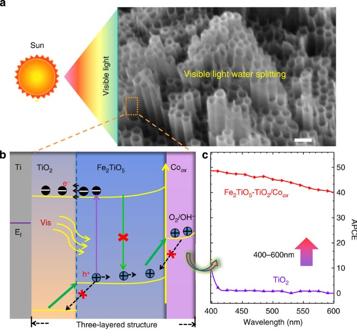These features correspond to the spectral characteristics of the iron titanate. Figure 1: Photoanode architecture and photoelectrochemical reaction mechanism. (a) Schematic of the sunlight irradiation on the composite Fe2TiO5-TiO2/Cooxnanotube-arrayed photoanode. Scale bar, 200 nm. (b) Schematic of the composite photoanode architecture and solar water oxidation mechanism, and (c) the resulting quantum efficiency of the photoanode.Ef, Fermi level. The model only represents the idealized electronic structure alignment of the composite photoanode. Figure 1: Photoanode architecture and photoelectrochemical reaction mechanism. ( a ) Schematic of the sunlight irradiation on the composite Fe 2 TiO 5 -TiO 2 /Co ox nanotube-arrayed photoanode. Scale bar, 200 nm. ( b ) Schematic of the composite photoanode architecture and solar water oxidation mechanism, and ( c ) the resulting quantum efficiency of the photoanode. E f , Fermi level. The model only represents the idealized electronic structure alignment of the composite photoanode. Full size image Figure 2: Morphology and structural properties of the samples. ( a , b ) Scanning electron microscopy and and ( c ) high-resolution TEM images for TiO 2 /Fe-contained/Co ox nanotube arrays. Scale bars, 200, 200, 5 and 100 nm, ( a , b , c and inset of c , respectively). ( d ) X-ray diffraction patterns for pure TiO 2 , Fe 2 TiO 5 reference sample and as-deposited TiO 2 /Fe-contained nanotube arrays, and grazing incidence X-ray diffraction patterns for the annealed TiO 2 /Fe-contained nanotube arrays. The standard card (PCPDF 76-1158) for orthorhombic Fe 2 TiO 5 is shown for reference. ( e ) Raman spectra for TiO 2 , TiO 2 /Fe-contained nanotube-arrayed photoanodes and reference Fe 2 TiO 5 (ref.). ( f ) Fe K -edge EXAFS FTs of k 3 χ ( k ) functions for TiO 2 /Fe-contained/Co ox . The empty circles show the fitting results. The Fe K -edge spectra for Fe 2 O 3 and Ti K -edge spectra for TiO 2 and Fe 2 TiO 5 (ref.) are shown for comparison. The reference Fe 2 TiO 5 (ref.) sample in d , e and f was synthesized by solid-state reaction method. Full size image Fe K -edge X-ray absorption fine structure (XAFS) spectroscopy that is sensitive to the local environment around a specific atom [22] is also employed to confirm the formation of Fe 2 TiO 5 in the TiO 2 /Fe-contained/Co ox nanotube arrays. First, the formation of Fe 2 O 3 can be ruled out, as the k 3 χ ( k ) oscillation shape and the corresponding Fourier transform (FT) curve ( Fig. 2f and Supplementary Fig. 6 ) of the sample are quite different from that of Fe 2 O 3 . Moreover, the positions (around 2.55 and 3.21 Å) of Fe–Ti coordination peaks in the FT curve of the sample are significantly lower than that of Ti–Ti1 and Ti–Ti2 peaks for TiO 2 , implying that the Fe atoms do not simply substitute for Ti in anatase TiO 2 . Furthermore, we show the FT spectrum at Fe K -edge for a reference compound Fe 2 TiO 5 in Fig. 2f . It can be found that the three FT peaks of the TiO 2 /Fe-contained/Co ox are well consistent with the spectrum of Fe 2 TiO 5 reference, indicating that the Fe-containing middle layer is truly in the form of the iron titanate Fe 2 TiO 5 . Moreover, the nominal thickness of Co layer is estimated as 0.5–1.0 nm, and Co K -edge XAFS measurements confirm the presence of short-range six-coordinated Co-based catalyst (Co ox ) on the surface of Fe 2 TiO 5 -TiO 2 ( Supplementary Fig. 7 ). Photoelectrochemical performance To investigate the photoelectrochemical performances of the Fe 2 TiO 5 -TiO 2 /Co ox nanotube-arrayed architecture, its quantum efficiency was measured and shown in Fig. 3a . For reference, the efficiencies of TiO 2 , TiO 2 /Co ox and Fe 2 O 3 nanotube-arrayed photoanodes are also displayed. The incident photon-to-current efficiency (IPCE, see Fig. 3a and Supplementary Note 1 ) curve shows that the Fe 2 TiO 5 -TiO 2 /Co ox nanotube array-based photoanode possesses a high IPCE of about 40% at the visible light wavelength of 475 nm, and it remains robust at longer wavelength (over 10% at 620 nm). In contrast, the efficiencies of both of the pristine TiO 2 - and Co ox -coated nanotubes are similar and extremely low, and Fe 2 O 3 nanotube ( Fig. 3 and Supplementary Figs 8 and 9 ) also has a low photon-to-current efficiency of <10%, which is in consistence with previous reports [23] . 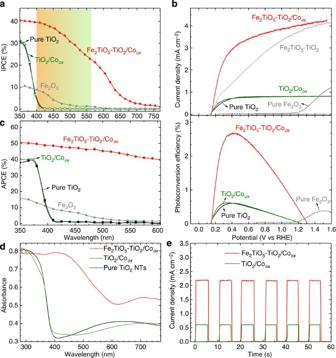Figure 3: Optical absorption and photoelectrochemical performance of the samples. (a) IPCE curves (measured at 0.4 V versus RHE for pure TiO2, TiO2/Cooxand Fe2TiO5-TiO2/Coox, and at 1.23 V versus RHE for Fe2O3). (b) Upper panel: dark current (dash lines) and photocurrent (solid lines) densities; lower panel: photoconversion efficiencies. (c) APCE curves of pure TiO2, TiO2/Coox, Fe2TiO5-TiO2/Cooxand Fe2O3photoanodes in 1 M KOH. (d) Ultraviolet-visible spectra of pure TiO2, TiO2/Cooxand Fe2TiO5-TiO2/Cooxsamples. (e) Transient photocurrent curves for TiO2/Cooxand Fe2TiO5-TiO2/Cooxphotoanodes performed with chopped light at 0.3 V versus RHE in 1 M KOH. Figure 3b shows a high current density of 4.1 mA cm −2 for the Fe 2 TiO 5 -TiO 2 /Co ox photoanode at 1.23 V versus RHE. In particular, the photocurrent onset potential of 0.18 V versus RHE corresponds to a small external bias of 0.2 V, which is significantly lower than that of narrow-bandgap Fe 2 O 3 (~1.0 V for pristine Fe 2 O 3 and ~0.7 V for Fe 2 O 3 modified with cocatalyst), resulting in a large total photoconversion efficiency of 2.7% ( Fig. 3b and Supplementary Note 2 ). The photocurrent is almost not degraded within 2 h ( Supplementary Figs 10 and 11 ), confirming the photoelectrochemical stability of the composite photoanode architecture. The saturated photocurrent of the composite photoanode is able to reach 4.2 mA cm −2 , which is comparable to that of recent FeOOH/NiOOH dual layer modified nanoporous BiVO 4 photoanode [24] and is noticeably higher than those of using pure metal oxides as visible light photon absorber [25] , [26] , [27] . Figure 3: Optical absorption and photoelectrochemical performance of the samples. ( a ) IPCE curves (measured at 0.4 V versus RHE for pure TiO 2 , TiO 2 /Co ox and Fe 2 TiO 5 -TiO 2 /Co ox , and at 1.23 V versus RHE for Fe 2 O 3 ). ( b ) Upper panel: dark current (dash lines) and photocurrent (solid lines) densities; lower panel: photoconversion efficiencies. ( c ) APCE curves of pure TiO 2 , TiO 2 /Co ox , Fe 2 TiO 5 -TiO 2 /Co ox and Fe 2 O 3 photoanodes in 1 M KOH. ( d ) Ultraviolet-visible spectra of pure TiO 2 , TiO 2 /Co ox and Fe 2 TiO 5 -TiO 2 /Co ox samples. ( e ) Transient photocurrent curves for TiO 2 /Co ox and Fe 2 TiO 5 -TiO 2 /Co ox photoanodes performed with chopped light at 0.3 V versus RHE in 1 M KOH. Full size image The APCE curves in Fig. 3c show that a highly efficient visible photoelectrochemical conversion with large quantum efficiencies has been realized when Fe 2 TiO 5 is incorporated in the nanotube-arrayed photoanode ( Supplementary Note 3 ). Moreover, the quantum efficiencies keep almost steady at a high level (45–50%) in the whole absorption range. Moreover, the Fe 2 TiO 5 -containing nanotube arrays with the length up to several micrometres ensure a substantial visible light absorption ( Fig. 3d ). Hence, our deliberately designed composite structure successfully overcomes low quantum efficiency limits of only a few per cent for transforming deep-visible photons to current by pristine oxide semiconductor photoanodes. In addition, the Fe 2 TiO 5 -containing photoanode combines the advantages of substantial optical absorption of narrow-bandgap Fe 2 O 3 and a low external bias of wide-bandgap TiO 2 to drive solar water oxidation. Together with the intrinsic merits of anticorrosion and cheapness of transition metal oxides, this composite system has shown its great potential as a practical photoelectrochemical material [28] . For a typical compact n-type semiconductor thin film photoanode, the magnitude of photocurrent corresponds to the number of photogenerated holes that react on the electrode surface. In general, it is determined by the competition of carriers migration and recombination [29] . To further investigate this competition in the Fe 2 TiO 5 -TiO 2 photoanode, the energy band positions are first analysed under scrutiny. Mott–Schottky plot and J 2 ∝ ( V − V fb ) relationship are usually used to identify the CBM position of n-type semiconductor electrode. As shown in Supplementary Fig. 12 , the flat band potentials of TiO 2 and Fe 2 TiO 5 are within 0.05 V difference and located at about 0.18 and 0.23 V versus RHE, respectively. Thus, the CBM positions are about 0 V versus RHE, which ensures the electron exchange between the two components. Considering the bandgap energy from the ultraviolet–visible absorption spectra, it is concluded that the valence band maximum (VBM) position of Fe 2 TiO 5 is about 1.0 eV above that of TiO 2 . The energy level of Co-layer catalyst identified as the redox potential is about 1.6 V versus RHE ( Supplementary Fig. 13 ). As a result, a gradient band structure forms, in which the interface between Fe 2 TiO 5 /TiO 2 makes the photoholes only transfer from the valence bands of Fe 2 TiO 5 to Co ox , while the electrons can migrate from the conduction bands of Fe 2 TiO 5 to TiO 2 ( Fig. 1b ). Meanwhile, the interface of Fe 2 TiO 5 /Co ox could timely trap the holes and transfer them onto the surface active sites because of its strong ability of absorbing holes. Hence, the hole–electron separation interface introduced by Fe 2 TiO 5 can well direct the transfer of hole carriers through the vectorial hole-transfer channel to reach the tube wall ( Fig. 1 and Supplementary Fig. 14 ). Indeed, the energy gradient of molecular orbitals can regulate charge transfer path on the molecular and semiconductor interface of dye-sensitized solar cells [30] . This Fe 2 TiO 5 -containing composite nanotube structure could alter the competition of carriers migration and recombination in two aspects: (1) the visible-light-generated holes are within 2 nm distance from the tube wall, which greatly shortens the diffusion layer width ( L ); and (2) the quick separation of holes and electrons from Fe 2 TiO 5 /TiO 2 interface could increase the photocarriers lifetime and diffusion length ( L pc ). From the APCE results in Figs 1c and 3c , it can be seen that the photons with wavelength of 620 nm (close to the absorption edge for Fe 2 TiO 5 -TiO 2 /Co ox ) could be effectively converted. In contrast, the effective photon-to-current conversion wavelength for pristine Fe 2 O 3 is up to about 500 nm, corresponding to an energy lower than the absorption edge of Fe 2 O 3 . This is presumably due to the inefficient separation and transportation of the low-energy carriers excited by the high-wavelength photons near the absorption edge [31] . Our quantum efficiency measurement for pristine Fe 2 O 3 nanotube photoanode is performed under 1.23 V versus RHE. It was reported that at a higher applied potential of 1.53 V versus RHE, the IPCE value of nanostructured Fe 2 O 3 photoanodes can increase to 45% in the 300–450 nm wavelength range [32] . Another point to note is that the performance of the composite structure is gradually decreased with increasing thickness of Fe 2 TiO 5 layer ( Supplementary Fig. 15 ). This suggests that the carrier-transport-guide effect of the hole–electron separation interface is significantly affected as the thickness of Fe 2 TiO 5 layer approaches the diffusion length, which is presumably responsible for the low photoelectrochemical performance of bulk Fe 2 TiO 5 photocatalyst [33] . On the other hand, decreasing the Fe 2 TiO 5 layer thickness would reduce the optical absorption. Therefore, the nominal 2 nm thickness of Fe 2 TiO 5 layer is optimized for achieving maximum visible-light conversion efficiency via the hole–electron separation interface. To validate the impact of vectorial hole-transfer channel on L and L pc , the electrochemical impedance spectroscopy (EIS) measurements are performed and shown in Fig. 4a . For nanostructure electrode with particle size sufficiently small (<10 nm), electromigration from band bending is likely to be negligible and transmission line model of EIS is suitable to evaluate the charge diffusion characteristics [34] , [35] . However, for the nanotube morphology electrode it becomes more complicated, as the geometry can be viewed as a combination of the characteristic nanostructure size in the radial direction with a macroscopic continuous pathway in the axial direction. Moreover, it is obvious that the diffusion photocurrent would be dominant ( Supplementary Fig. 16 ), which is also indicated by the large photocurrent of Fe 2 TiO 5 -TiO 2 /Co ox at the flat band potential. Based on these facts, an equivalent circuit has been developed and displayed in the inset of Fig. 3a , where the series resistance represents the charge carrier diffusion along the axial direction, while the parallel resistance stands for the charge carrier diffusion along the radial direction ( Supplementary Note 4 and Supplementary Fig. 17 ). It can be found that the transmission impedance is significantly reduced, probably because the weight of equivalent circuits is transferred from series connection to parallel connection. The L pc / L increases by more than ten times compared with that of TiO 2 ( Fig. 4b ) and Fe 2 O 3 ( Supplementary Fig. 18 ), when the Fe 2 TiO 5 layer is introduced in the nanotubes. These results indicate an enhanced charge carrier transfer ability in the composite structure ( Fig. 1b ), which is due to the carrier separation interface of Fe 2 TiO 5 /TiO 2 that has successfully separated the electrons and holes to the different diffusion regions of TiO 2 layer and Fe 2 TiO 5 layer, respectively. This leads to a maximized gradient of carrier distribution and results in the regulated carriers distribution and the prolonged carriers lifetime. Moreover, the transient photocurrent measurements in Fig. 3e show that the steady-state photocurrent densities of Fe 2 TiO 5 -TiO 2 /Co ox photoanode are significantly enhanced relative to those of parent TiO 2 -based photoanodes. Evidently, there are no spikes within the first second of irradiation in the transient photocurrent spectrum of Fe 2 TiO 5 -TiO 2 /Co ox , suggesting that the hole transfer bottlenecks from the interior to outside of Fe 2 TiO 5 -TiO 2 /Co ox nanotubes is resolved [36] . Hence, these results demonstrate an anisotropic charge carrier transfer character in the composite structure, which is further confirmed by the sequential injection of negative charges by the overlayer ( Supplementary Note 5 ). Benefiting from the vectorial hole-transfer channel, an effective collection of charge carriers excited by the visible light is realized in the composite structure. 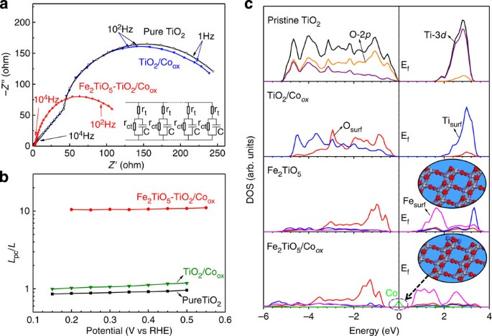Figure 4: Electrochemical impedance properties and electronic structure modelling. (a) Electrochemical impedance spectra measured for the samples,Z’ andZ” are the real and imaginary parts of impedance. The inset shows the equivalent circuit. (b) Calculated carrier diffusion lengths for the pristine TiO2, TiO2/Cooxand Fe2TiO5-TiO2/Cooxnanotube films. (c) Calculated electronic structures for pristine TiO2, TiO2/Cooxand Fe2TiO5-TiO2/Cooxmodels. The insets show the model structures used for calculations. Figure 4: Electrochemical impedance properties and electronic structure modelling. ( a ) Electrochemical impedance spectra measured for the samples, Z ’ and Z ” are the real and imaginary parts of impedance. The inset shows the equivalent circuit. ( b ) Calculated carrier diffusion lengths for the pristine TiO 2 , TiO 2 /Co ox and Fe 2 TiO 5 -TiO 2 /Co ox nanotube films. ( c ) Calculated electronic structures for pristine TiO 2 , TiO 2 /Co ox and Fe 2 TiO 5 -TiO 2 /Co ox models. The insets show the model structures used for calculations. Full size image The oxidation activity of the holes that transport to surface is intimately related to the electronic structure of the surface states. Figure 4c shows the calculated density of states for the different structural configurations. For pristine TiO 2 and Fe 2 TiO 5 , the Fermi level locates in the middle of the vacant bandgap, in line with the band structure character of ideal semiconductor. It can be seen that the Co ox can hardly change the energy states of surface Ti (Ti surf ) and O (O surf ) atoms of TiO 2 (see the second panel of Fig. 4c ). However, as Co ox coupled with Fe 2 TiO 5 , a gap state across the Fermi level is formed, because of the interaction between the Co ox (green curve) and surface O (red curve) atoms as shown in the bottom panel of Fig. 4c . The gradient energy level of the highest occupied energy state confirms the vectorial transfer of charges in the nanotube. Meanwhile, a half-empty energy band of Co ox is formed in the gap (denoted by the arrow in Fig. 4c ). Speaking in general, the catalytic activity of photoanode is strongly dependent on the property of surface energy states, especially the d orbital states that directly participate in the water redox reaction [37] . The half-empty energy state of surface O and Co can strongly increase the binding of the initial product OH of water splitting and overcome the reaction barrier, resulting in an enrichment of OH on the Fe 2 TiO 5 /Co ox surface. This makes the required bias of Fe 2 TiO 5 /Co ox surface for water cleavage reduce to 200 mV, which matches well with the hole energy of Fe 2 TiO 5 . It is worth noting that for Fe 2 TiO 5 -TiO 2 nanotube arrays, the VBM position is upshifted by 1.0 eV compared with pure TiO 2 . The overpotential of photogenerated holes at the VBM is then greatly decreased and thus it is not sufficient for the water oxidation, which is confirmed by the photocurrent curve of Fe 2 TiO5-TiO 2 in Fig. 3b . The photocurrent value of Fe 2 TiO 5 -TiO 2 approaches that of Fe 2 TiO 5 -TiO 2 /Co ox at higher overpotential, indicating a similar diffusion efficiency ( Supplementary Discussion ). In addition to the highly efficient hole transfer via the vectorial hole-transfer channel, both ultraviolet and visible light excited holes can efficiently catalyse water oxidation through the Co ox catalyst. In summary, we develop a simple strategy to fabricate a new pseudobrookite Fe 2 TiO 5 material deposited on the vertically oriented TiO 2 nanotube arrays, for the efficient separation and transportation of low-energy visible-light-excited charge carriers. The grazing incidence X-ray diffraction, Raman and XAFS techniques indicate the formation of Fe 2 TiO 5 layers on the TiO 2 nanotube arrays. The quantum efficiency measurements demonstrate that this Fe 2 TiO 5 -containing nanotube arrays with a low onset potential of ~0.2 V exhibit a sustainably high quantum efficiency of >40% from ultraviolet to 600 nm with a total energy conversion efficiency of 2.7%. Combining ultraviolet–visible absorption, EIS and first-principles density functional theory calculations, the high visible photoelectrochemical performance of this composite structure can be attributed to the anisotropic charge carrier transport and reduced charge carrier transfer resistance. Moreover, the vertically aligned nanotube arrays with huge specific surface areas and superior transport property offer a well-behaving architecture, which in turn promotes the transfer of the visible-light-excited photoholes to the photocatalyst surface to participate in water redox reactions. By extending the optical absorption towards far visible regions, the overall photoelectrochemical efficiencies of these processes and/or devices are expected to be further enhanced. To overcome the deficiency of back-side illumination on the photoelectrode, the base of TiO 2 nanotube arrays grown on fluorine-doped tin oxide glass substrate has been proposed [38] , where more efficient front-side illumination could be realized. Our design may open up opportunities to modify the semiconductor oxides towards high photoconversion efficiency for practical photochemical applications. Materials Titanium foil (0.25 mm thickness, 99.99% trace metals basis, Aldrich) was used for electrochemical anodization. Ethylene glycol, ammonium fluoride, ferric nitrate, cobalt nitrate and potassium phosphate (all from Aldrich) were used as precursors. Synthesis of TiO 2 nanotube-arrayed photoanodes The Fe 2 TiO 5 layer supported on the highly ordered TiO 2 nanotube arrays was prepared by an electrochemical deposition in combination with post-annealing method. First, the TiO 2 nanotube arrays were prepared by the electrochemical anodization in a NH 4 F organic electrolyte with optimized performance. Briefly, the pure titanium foils were ultrasonically cleaned with acetone, ethanol and deionized water, followed by drying under a nitrogen stream. Then, the Ti foils were immersed in a mixed ethylene glycol solution of 0.35 wt.% NH 4 F and 2 vol.% deionized water, and subjected to a constant potential (60 V) at room temperature in a two-electrode configuration with titanium foil as the working electrode and platinum mesh as the counter electrode. An Fe 2 O 3 layer was subsequently electrodeposited onto TiO 2 nanotubular array film in a 5-mM Fe(NO 3 ) 3 solution at −0.6 V versus AgCl/Ag. Then, the heterojunction products were annealed at 550 °C for 2 h in ambient air to obtain Fe 2 TiO 5 /TiO 2 composite bilayer. For the Co ox deposition, the photoanode was submerged in an electrolyte solution of 25 mM Co(NO 3 ) 2 in 0.1 M K 2 SO 4 (pH 7.0) and a bias of 1.6 V (versus RHE) was applied for 3 min. Electrochemical impedance spectroscopy measurement Electrochemical impedance spectra measurements of TiO 2 -based photoanodes were performed with an electrochemical workstation (Model CHI760D, CH instruments, Inc., Austin, TX) with a three-electrode system, which was operated with the TiO 2 nanotube array films as anode, platinum mesh as cathode and Ag/AgCl as reference electrode. The spectra were measured at various forward bias voltages (from 0.15 to 0.5 V versus RHE) in the frequency range of 0.1 Hz–1 MHz with oscillation potential amplitudes of 10 mV at room temperature. XAFS measurement and data analysis The Fe K -edge XAFS spectroscopy were recorded in the fluorescence mode at U7C beamline in the National Synchrotron Radiation Laboratory, China, 1W1B beamline of Beijing Synchrotron Radiation Facility, China, and BL14W1 beamline of Shanghai Synchrotron Radiation Facility, China. The acquired extended XAFS (EXAFS) data were processed according to the standard procedures using the ATHENA module implemented in the IFEFFIT software packages. The EXAFS χ ( k ) spectra were obtained by subtracting the post-edge background from the overall absorption and then normalized with respect to the edge-jump step. Subsequently, k 3 -weighted χ ( k ) data in the k -space ranging from 2.8 to 11.8 Å −1 were Fourier transformed to real ( R ) space using a hanning windows (d k =1.0 Å −1 ) to separate the EXAFS contributions from different coordination shells. Density functional theory calculation details The first-principles density functional theory+ U calculations were performed using a plane wave basis set with the projector augmented plane-wave method [39] , [40] , [41] , [42] . The exchange-correlation interaction was described within the generalized gradient approximation in the form of PW91 (refs 43 , 44 ). The energy cutoff was set to 400 eV and the atomic positions were allowed to relax until the energy and force were <10 −4 eV and 10 −3 eV Å −1 , respectively. We used a 2 × 2 two-dimensional unit cells of anatase TiO 2 (101) and Fe 2 TiO 5 (110) consisting of a four-trilayer slab and a vacuum region of 12 Å to mimic the TiO 2 and Fe 2 TiO 5 tube surfaces. How to cite this article: Liu, Q.H. et al . Aligned Fe 2 TiO 5 -containing nanotube arrays with low onset potential for visible-light water oxidation. Nat. Commun. 5:5122 doi: 10.1038/ncomms6122 (2014).